A structural basis for streptomycin-induced misreading of the genetic code During protein synthesis, the ribosome selects aminoacyl-transfer RNAs with anticodons matching the messenger RNA codon present in the A site of the small ribosomal subunit. The aminoglycoside antibiotic streptomycin disrupts decoding by binding close to the site of codon recognition. Here we use X-ray crystallography to define the impact of streptomycin on the decoding site of the Thermus thermophilus 30S ribosomal subunit in complexes with cognate or near-cognate anticodon stem–loop analogues and messenger RNA. Our crystal structures display a significant local distortion of 16S ribosomal RNA induced by streptomycin, including the crucial bases A1492 and A1493 that participate directly in codon recognition. Consistent with kinetic data, we observe that streptomycin stabilizes the near-cognate anticodon stem–loop analogue complex, while destabilizing the cognate anticodon stem–loop analogue complex. These data reveal how streptomycin disrupts the recognition of cognate anticodon stem–loop analogues and yet improves recognition of a near-cognate anticodon stem–loop analogue. The bacterial ribosome is a major target of antibiotic inhibitors of protein synthesis. The solution of cocrystal structures of ribosome–antibiotic complexes has greatly expanded our understanding of antibiotic modes of action and has also provided mechanistic insights into the individual steps of protein synthesis that are impacted by these drugs [1] . While some antibiotics act as competitive inhibitors of transfer RNA substrates of the ribosome, others act by perturbing ribosome conformation. The latter is especially true of the aminoglycoside antibiotic streptomycin, which severely impairs the ribosome’s ability to accurately decode messenger RNA. Although investigation into the mode of action of streptomycin has been the subject of intense scrutiny for decades [2] , the description of streptomycin action remains incomplete. Much of what we know about its mechanism of action comes from observations of the phenotypic behaviour of resistant mutants and from the observed effects of the drug on decoding by ribosomes in vitro . Streptomycin causes phenotypic suppression of nonsense mutations in vivo [3] and leucine misincorporation in poly-U-directed poly-phenylalanine synthesis in vitro [4] , whereas streptomycin-resistant mutants are hyperaccurate as indicated by restriction of readthrough of leaky nonsense mutations [5] . More recent, pre-steady-state kinetic experiments have dissected the relationship between streptomycin and guanosine triphosphate (GTP) hydrolysis by EF-Tu [6] . In the absence of streptomycin, GTP hydrolysis is very fast for cognate codon complexes and much slower for near-cognate complexes, thereby driving tRNA selection in the forward direction and allowing a proofreading step. Streptomycin reduces the rate of GTPase activation for cognate codons and increases the rate of GTPase activation for near-cognate codons resulting in similar activation rates and loss of ribosomal selectivity [7] . This is distinct from the effect of another error-inducing aminoglycoside, paromomycin, which specifically increases activation with near-cognate substrates [6] . The streptomycin-binding site, as determined by X-ray crystallography [8] , comprises 16S ribosomal RNA helices 1, 18, 27 and 44, and ribosomal protein S12. On the basis of the close interaction of streptomycin with the decoding site and the shoulder region, it was proposed that streptomycin induces miscoding by stabilizing the closed conformation of the 30S subunit, thereby increasing the rate of GTPase activation of EF-Tu in the presence of codon–anticodon mismatches [8] . Paromomycin binds to the decoding site but its binding site does not overlap that of streptomycin [8] . It forces the bases A1492 and A1493 to flip out of helix 44 and interact with the minor groove of the codon–anticodon minihelix, as they do upon cognate codon recognition as part of an induced-fit mechanism. This re-positioning facilitates formation of a closed conformation in the ribosome (indicated by a shift of helix 18 and ribosomal protein S12 in the shoulder domain), resembling the cognate decoded state even with near-cognate tRNA substrates [8] , [9] . The antibiotic contributes part of the energy required to activate GTP hydrolysis by EF-Tu and even increases GTPase activation in the presence of codon–anticodon mismatches. Although the crystal structure of paromomycin bound to the 30S subunit has been reported in the absence of other antibiotics [9] , the only streptomycin-bound 30S subunit structure also contained paromomycin and spectinomycin [8] . Also lacking are any ribosome-streptomycin structures in the presence of either cognate or near-cognate tRNA–mRNA complexes. We have determined 30S subunit-streptomycin cocrystal structures, allowing us to distinguish the conformational effects of streptomycin from those of other antibiotics. We also determined 30S subunit-streptomycin structures in decoding complexes with cognate or near-cognate anticodon stem–loop analogues (ASLs). Rather than adopting the closed conformation, streptomycin shifts the decoding site region of 16S rRNA helix 44 laterally in the direction of ribosomal protein S12 and helix 18, without the flipping out of A1492 and A1493 from helix 44 as seen with paromomycin. By pre-organizing the decoding site in a previously unobserved conformation, streptomycin destabilizes cognate ASL–mRNA complexes while stabilizing near-cognate complexes. This provides a structural framework for interpretation of previous kinetic experiments. 30S subunit structure determination To study the structural impact of streptomycin, we purified and crystallized Thermus thermophilus 30S subunits in space group P4 1 2 1 2 as described previously [10] , [11] . We generated complexes with streptomycin, hexa-uridine mRNA, and cognate ASL Phe GAA (data set Phe, Protein Data Bank (PDB) accession code 4DR5 ) or near-cognate ASLs (ASL Leu2 GAG , data set Leu, PDB accession code 4DR6 , and ASL Ser GGA , data set Ser, PDB accession code 4DR7 ) by soaking these compounds into 30S subunit crystals. Seven X-ray diffraction data sets were collected with resolution ranging from 3.25 to 3.95 Å ( Supplementary Table S1 ). Clear difference electron density was visible in the streptomycin-binding site for each streptomycin soaking experiment ( Fig. 1 ). Streptomycin binds adjacent to the 30S decoding site, forming hydrogen bonds and salt bridges with backbone phosphates of 16S rRNA residues U14 in helix 1, C526 and G527 in helix 18, A914 in helix 27, and C1490 and G1491 in helix 44. Lysine residues 42 and 87 ( Escherichia coli numbering is used throughout) from ribosomal protein S12 may form additional hydrogen bonds although electron density is not defined for these protein side chains. 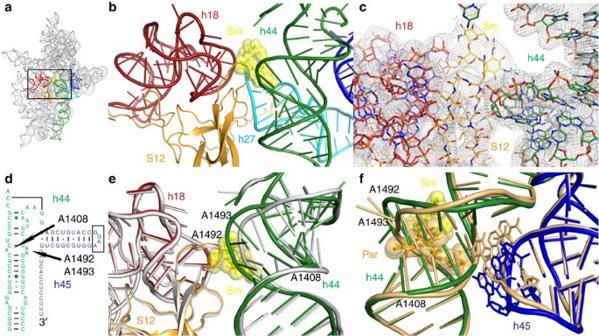Figure 1: Conformational changes upon binding of streptomycin to the 30S subunit. (a) Cartoon representation of the 16S rRNA seen from the subunit interface. The region shown inbis indicated with a black rectangle. (b) Streptomycin-binding site in the 30S subunit. Streptomycin is shown as yellow sticks and spheres. Helix 44 is shown as dark-green cartoon, helix 18 is coloured in red, helix 27 in cyan, helix 45 in blue and protein S12 in orange. (c) Final σA-weighted m2Fo-dFcelectron density map of the streptomycin-binding site contoured at 1σ. (d) Secondary structure diagram of the decoding site region in helix 44 and of the helix 45 tetraloop (indicated with a box). (e) Conformational changes in the decoding site upon streptomycin binding. The streptomycin-bound 30S structure is shown superimposed onto the apo 30S structure shown in light grey. (f) Comparison of the two helix 45 tetraloop conformations induced by streptomycin (data set Strep, PDB accession code4DR3) and paromomycin (data set Par, PDB accession code4DR2, coloured in light orange). Figure 1: Conformational changes upon binding of streptomycin to the 30S subunit. ( a ) Cartoon representation of the 16S rRNA seen from the subunit interface. The region shown in b is indicated with a black rectangle. ( b ) Streptomycin-binding site in the 30S subunit. Streptomycin is shown as yellow sticks and spheres. Helix 44 is shown as dark-green cartoon, helix 18 is coloured in red, helix 27 in cyan, helix 45 in blue and protein S12 in orange. ( c ) Final σ A -weighted m2F o -dF c electron density map of the streptomycin-binding site contoured at 1σ. ( d ) Secondary structure diagram of the decoding site region in helix 44 and of the helix 45 tetraloop (indicated with a box). ( e ) Conformational changes in the decoding site upon streptomycin binding. The streptomycin-bound 30S structure is shown superimposed onto the apo 30S structure shown in light grey. ( f ) Comparison of the two helix 45 tetraloop conformations induced by streptomycin (data set Strep, PDB accession code 4DR3 ) and paromomycin (data set Par, PDB accession code 4DR2 , coloured in light orange). Full size image To compare the impact of streptomycin with that of paromomycin, we performed a control experiment with cognate ASL Phe GAA and mRNA in the presence of paromomycin (data set MAP, PDB accession code 4DR4 ). We observed well-defined electron density for the ASL Phe GAA and mRNA. Paromomycin stabilized the closed conformation of the 30S helix 18 in the ASL and mRNA-bound 30S structure, highly similar to previously published data. The root-mean-square deviation (rmsd) between all 16S rRNA phosphate atoms of our apo-30S structure and the equivalent PDB entry 1J5E (ref. 12 ) is 0.79 Å, and the rmsd between our MAP structure and PDB entry 1IBL [9] is 0.48 Å ( Supplementary Fig. S1 ). In comparison, the rmsds between open and closed 30S structures are 1.2 Å between the Apo and MAP data sets, and 0.97 Å between the analogous PDB entries 1J5E and 1IBL [9] , [12] , [13] . Because aminoglycosides are known for their RNA-binding properties, we explored the possibility of additional non-inhibitory binding sites for paromomycin by soaking experiments with higher concentrations of the antibiotic (800 μM). We observed multiple sites of difference electron density peaks large enough to be consistent with paromomycin molecules in both data sets ( Supplementary Fig. S2 ). The Phenix program package [14] automatically placed 17 and 18 paromomycin molecules into difference electron density maps of the Par and MAP data sets. Sixteen of these sites are occupied in both data sets, and eight molecules were placed in an identical orientation. Difference density peaks at these sites were not observed for other data sets. In contrast, we did not observe any secondary streptomycin-binding sites. Streptomycin restructures the 30S decoding site A comparison of the streptomycin-bound decoding site with the empty decoding site reveals that the antibiotic does not induce a conformational change in helix 18 (‘shoulder closure’, Fig. 1e and Supplementary Fig. S3 ). However, streptomycin does induce a lateral shift of helix 44 between C1490 and U1498, including the crucial bases A1492 and A1493 in the decoding site, by up to 3.5 Å. Thus, streptomycin reduces the distance between helices 18 and 44 but does so by distorting helix 44 instead of the shoulder helix 18. Unlike paromomycin, however, streptomycin does not induce A1492 and A1493 to flip out of the helix. An additional conformational change was observed upon streptomycin binding involving the interaction of helix 44 with the neighbouring helix 45. Analysis of electron density for the helix 45 tetraloop between G1516 and G1520 reveals two conformations. In the presence of the antibiotic paromomycin, the helix 45 tetraloop assumes an extended conformation and forms stabilizing hydrogen bonds with helix 44 (‘engaged’ conformation). In the presence of streptomycin, the same region retracts from helix 44 (‘disengaged’ conformation). This disengaged conformation is observed in data sets Strep and Leu ( Figs 1f and 2 ). Increased disorder in the neighbouring helix 24a accompanies disruption of the helix 45–helix 44 interaction, as indicated by the weakly defined electron density for this helix. Electron density for helix 45 in our apo 30S data set suggests the presence of both alternate conformations. Together, these data indicate that the helix 45 tetraloop region is dynamic in the apo 30S structure and forms a stable interaction (the engaged conformation) during decoding of cognate tRNAs. This engaged conformation is further stabilized by paromomycin, but destabilized by the conformational shift of helix 44 in the presence of streptomycin. 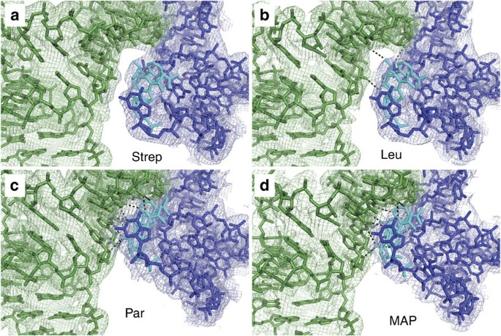Figure 2: Helix 45 conformation in four 30S crystal structures. Final σA-weighted 2mFo-DFcelectron density contoured at 1σ is shown for helix 44 coloured in green and helix 45 coloured in blue with A1518 and A1519 coloured in cyan. (a) streptomycin bound, (b) streptomycin, mRNA and ASLLeu2GAG, (c) paromomycin and (d) paromomycin, mRNA and ASLPheGAA. Figure 2: Helix 45 conformation in four 30S crystal structures. Final σ A -weighted 2mF o -DF c electron density contoured at 1σ is shown for helix 44 coloured in green and helix 45 coloured in blue with A1518 and A1519 coloured in cyan. ( a ) streptomycin bound, ( b ) streptomycin, mRNA and ASL Leu2 GAG , ( c ) paromomycin and ( d ) paromomycin, mRNA and ASL Phe GAA . Full size image Effects of streptomycin on decoding complexes To examine the effect of streptomycin on decoding, we soaked 30S crystals with hexa-uridine mRNA and either cognate ASL Phe GAA , near-cognate ASL Leu2 GAG (first position mismatch) or ASL Ser GGA (second position mismatch). All soaking experiments were performed using analogous conditions, but only the electron density for the near-cognate ASL Leu2 GAG was well defined for the base-pairing nucleotides in the mRNA and ASL ( Fig. 3a ). Because of the weak electron density for soaking experiments with the ASL Phe GAA and ASL Ser GGA , only the data set for the near-cognate ASL Leu2 GAG was used for further structural analysis. 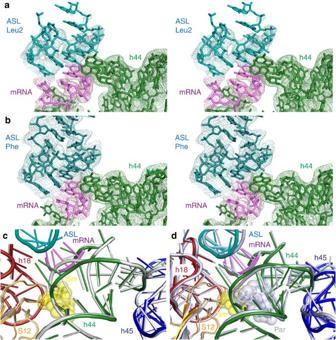Figure 3: Decoding of near-cognate ASLLeu2GAGin the presence of streptomycin. (a) σA-weighted 2mFo-DFcelectron density (contoured at 1σ) for the ASLLeu2GAG, mRNA, and helix 44 in the presence of streptomycin. ASL, mRNA and helix 44 are coloured in blue, violet and green, respectively. (b) σA-weighted 2mFo-DFcelectron density (contoured at 1σ) for the ASLPheGAA, mRNA and helix 44 in the presence of paromomycin. (c) Conformational changes (and compensatory shift of the phosphate backbone) of bases A1492 and A1493 in the presence of the near-cognate ASLLeu2GAG, mRNA and streptomycin (coloured as inFig. 1) compared with the streptomycin-bound 30S subunit (coloured in light grey). (d) Comparison of near-cognate ASLLeu2GAGposition in the presence of streptomycin (coloured as before) with cognate ASLPheGAAin the presence of paromomycin (MAP data, PDB accession code4DR4, coloured in grey). Figure 3: Decoding of near-cognate ASL Leu2 GAG in the presence of streptomycin. ( a ) σ A -weighted 2mF o -DF c electron density (contoured at 1σ) for the ASL Leu2 GAG , mRNA, and helix 44 in the presence of streptomycin. ASL, mRNA and helix 44 are coloured in blue, violet and green, respectively. ( b ) σ A -weighted 2mF o -DF c electron density (contoured at 1σ) for the ASL Phe GAA , mRNA and helix 44 in the presence of paromomycin. ( c ) Conformational changes (and compensatory shift of the phosphate backbone) of bases A1492 and A1493 in the presence of the near-cognate ASL Leu2 GAG , mRNA and streptomycin (coloured as in Fig. 1 ) compared with the streptomycin-bound 30S subunit (coloured in light grey). ( d ) Comparison of near-cognate ASL Leu2 GAG position in the presence of streptomycin (coloured as before) with cognate ASL Phe GAA in the presence of paromomycin (MAP data, PDB accession code 4DR4 , coloured in grey). Full size image In the 30S complex structure with bound near-cognate ASL Leu2 GAG , mRNA, and streptomycin, we observed clear electron density for A1492 and A1493 in their flipped-out conformation and for G530 in the anti conformation, indicating a bona fide decoding interaction of the near-cognate ASL. Compared with the 30S structure with only streptomycin bound, the distortion of the helix 44 backbone is largely reversed to accommodate the interaction of A1492 and A1493 with the codon–anticodon minihelix ( Fig. 3c ). As a result, the conformation of the decoding site with near-cognate ASL–mRNA in the presence of streptomycin approaches the conformation of the cognate ASL–mRNA in the presence of paromomycin ( Fig. 3d ). The distortion of helix 44 by streptomycin and the reversal of this distortion upon decoding of a near-cognate ASL are consistent with an improved recognition of near-cognate tRNAs and a reduced recognition of cognate tRNAs. Surprisingly, we identified an additional region of high difference electron density near the 3′ end of 16S rRNA that was consistent with a reorganization of the 16S 3′-tail and the formation of a Shine-Dalgarno-Anti-Shine-Dalgarno helix with a second molecule of ASL Leu2 GAG ( Supplementary Fig. S4 ). We observed this helix formation after soaking with near-cognate ASL Leu2 GAG and ASL Ser GGA but not with the cognate ASL Phe GAA . We note that the secondary structure of the near-cognate ASLs is weaker than that of the cognate ASL, which could have caused increased unfolding of the near-cognate ASLs and subsequent imperfect base-pairing of the unfolded ASLs with the 16S 3′-tail to form this Shine-Dalgarno-like interaction. In contrast to paromomycin, streptomycin does not stabilize 30S shoulder closure (a shift of helix 18, of the S12 Lys 42 loop, and of the ASL) even in the presence of cognate or near-cognate ASLs and mRNA ( Fig. 3d ). The absence of closure of helix 18 can also be visualized by plotting the distances between backbone phosphate atoms of two aligned 30S structures, as was done previously to visualize domain closure with cognate ASL in the presence of paromomycin ( Supplementary Fig. S3 , [13] ). Additionally, domain closure results in movements far from the decoding site, including a shift of the relative positions of ribosomal proteins S4 and S5. A change in the positions of proteins S4 and S5 in the streptomycin-bound structures was not observed, consistent with a lack of domain closure in the presence of streptomycin. Formation of helix 44–helix 45 contacts seen in paromomycin-bound structures is not observed in the presence of streptomycin. The helix 45 tetraloop remains disengaged in the presence of streptomycin after binding of near-cognate ASL and mRNA ( Fig. 3d ). Formation of the helix 44–45 contact may depend on proper orientation of helix 44, and the failure to interact may reflect the streptomycin-induced distortion of helix 44. In combination, these structures show that streptomycin destabilizes cognate complexes and stabilizes near-cognate complexes, unlike paromomycin, which acts primarily by stabilizing near-cognate complexes. Our observation that streptomycin and paromomycin influence ribosome structure in distinct ways is entirely consistent with pre-steady-state kinetic data showing that these drugs impact GTP hydrolysis in distinct ways. These data provide a structural framework for kinetic observations of the effects of these drugs on GTPase activation of EF-Tu [6] . In this study, our objective was to determine the structural basis for streptomycin-induced misreading of the genetic code. We produced X-ray crystal structures of 30S ribosomal subunits in complex with streptomycin and cognate or near-cognate ASLs. Streptomycin binds to a single site and induces a unique conformational change in the decoding site of the 30S subunit. In the presence of the antibiotic, binding of a near-cognate ASL is stabilized whereas binding of a cognate ASL is destabilized. The streptomycin-induced lateral shift of helix 44 in this study would appear to be sufficient to account for misreading but we cannot exclude the possibility that streptomycin also contributes to the energetics of ribosomal decoding by additional stabilization of near-cognate tRNAs in a closed 30S conformation. The binding site of streptomycin on the 30S subunit has been determined previously by X-ray crystallography in a triple complex together with paromomycin and spectinomycin [8] . In this complex, the helix 44 decoding region assumes a conformation similar to the paromomycin-only conformation, suggesting that the paromomycin-induced flipping out of A1492 and A1493 overrides the streptomycin-induced distortion of the helix 44 backbone. A dominant effect of paromomycin seems plausible considering that paromomycin occupies the apo position of A1492 and A1493, and displaces both bases whereas streptomycin only interacts with the backbone of bases C1490 and G1491. To compare the effects of streptomycin and paromomycin, we also obtained structures for apo 30S subunits and for 30S subunits in complex with paromomycin or mRNA/cognate ASL Phe GAA /paromomycin. These latter structures closely match analogous structures from the Ramakrishnan group [9] , [12] , [13] , although with higher concentrations of paromomycin, we observed multiple secondary binding sites for this antibiotic ( Supplementary Fig. S2 ). This observation is supported by a number of previous studies by others and has potential implications for in vitro ribosome studies in the presence of paromomycin [15] , [16] , [17] , [18] , [19] , [20] . However, the isolation of single-site paromomycin-resistance mutations [21] , [22] clearly shows that a single paromomycin-binding site is responsible for antibiotic activity. The multiple secondary bindings sites of this aminoglycoside antibiotic in structures presented here may overlap with sites occupied in vivo by polyamines. Further evidence to support the concept that the helix 44 decoding region is dynamic comes from 30S subunit crystal structures in complex with initiation factor (IF)1 or with the bacteriocin colicin E3. IF1 induces extensive shifts between bases C1490 and A1493 (ref. 23 ) and colicin E3 cleaves between bases A1493 and G1494 (ref. 24 ) while contacting structural elements that are involved in streptomycin binding [25] . Streptomycin restructures the decoding site in a manner that reduces the binding affinity of IF1 (ref. 26 ), and blocks the action of colicin E3 (ref. 27 ), providing independent evidence for streptomycin-induced conformational changes in the decoding site. Streptomycin stabilizes a near-cognate mismatch in the first position to a larger extent than the same mismatch in the second position or even the cognate interaction. The same preferential stabilization of the binding of ASL Leu2 GAG over ASL Ser GGA by paromomycin has been observed previously [13] , consistent with more efficient discrimination against near-cognate ASLs having mismatches in the second position [28] . A comparison of the placement of the near-cognate ASL Leu2 GAG with streptomycin and the cognate ASL Phe GAA without antibiotic (PDB entry 1IBM [9] ) confirms that streptomycin stabilizes the near-cognate ASL in a cognate-like overall conformation with small local changes to accommodate the mismatch ( Fig. 4a ). The first position mismatch in the near-cognate ASL causes a shift in A1493 of 16S rRNA and G36 of the ASL, whereas the mRNA bases remain in a similar position. A second comparison illustrates how 30S domain closure compacts the base-pairing interaction between ASL and mRNA, and stabilizes the A site tRNA on the 30S subunit. A superposition of our streptomycin/ASL/mRNA-bound 30S subunit structure in the open conformation with the same near-cognate ASL Leu2 GAG in the paromomycin-stabilized closed conformation (PDB entry 1N32, [13] ) shows conformational shifts of A1492/A1493, ASL, and of the mRNA to accommodate the first base mismatch ( Fig. 4b ). Analogous shifts of mRNA and tRNA positions can also be seen in comparison with recent crystal structures of 70S ribosomes with near-cognate tRNAs in the A site in the proofreading stage [29] . However, additional movements of the 30S head domain in the 70S ribosome and the use of a longer mRNA induce additional shifts in the codon–anticodon positions that preclude a detailed comparison with our results. Together these structural data show that conformational changes in the helix 44 region can occur independently of domain closure. This suggests that the formation of the tRNA–mRNA minihelix and conformational changes in helix 44 precede domain closure movements of the shoulder region and of the 30S head domain. 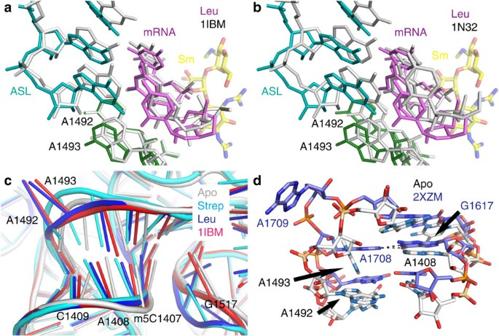Figure 4: Conformational flexibility in the 30S decoding site. (a) Comparison of decoding interactions for near-cognate ASLLeu2GAG(data set Leu, PDB accession code4DR6, coloured as before) with cognate decoding interactions (PDB accession code1IBMcoloured in grey9). (b) Data set Leu coloured as before compared to PDB accession code1N32(30S subunit in complex with near-cognate ASLLeu2GAG, mRNA, and paromomycin, coloured in grey13). Paromomycin-induced domain closure shifts the position of the near-cognate ASL, mRNA and A1492/A1493 when compared with the open, streptomycin stabilized interaction shown ina. (c) Restructuring of the helix 44 region by streptomycin. The position of bases C1407–C1409 opposite of A1492 and A1493 is shifted upon streptomycin binding both in the absence (cyan) and presence (blue) of ASL and mRNA when compared with the apo-30S structure (grey) or the cognate decoding structure PDB accession code1IBM(red). (d) Comparison of the helix 44 decoding region (coloured in white) with the eukaryotic 40S subunit fromTetrahymena thermophila(coloured in blue, PDB accession code2XZM33). A1708 (equivalent to A1492) forms a non-Watson–Crick base pair with G1617 (equivalent to A1408), while A1709 is flipped out of the helix. Figure 4: Conformational flexibility in the 30S decoding site. ( a ) Comparison of decoding interactions for near-cognate ASL Leu2 GAG (data set Leu, PDB accession code 4DR6 , coloured as before) with cognate decoding interactions (PDB accession code 1IBM coloured in grey [9] ). ( b ) Data set Leu coloured as before compared to PDB accession code 1N32 (30S subunit in complex with near-cognate ASL Leu2 GAG , mRNA, and paromomycin, coloured in grey [13] ). Paromomycin-induced domain closure shifts the position of the near-cognate ASL, mRNA and A1492/A1493 when compared with the open, streptomycin stabilized interaction shown in a . ( c ) Restructuring of the helix 44 region by streptomycin. The position of bases C1407–C1409 opposite of A1492 and A1493 is shifted upon streptomycin binding both in the absence (cyan) and presence (blue) of ASL and mRNA when compared with the apo-30S structure (grey) or the cognate decoding structure PDB accession code 1IBM (red). ( d ) Comparison of the helix 44 decoding region (coloured in white) with the eukaryotic 40S subunit from Tetrahymena thermophila (coloured in blue, PDB accession code 2XZM [33] ). A1708 (equivalent to A1492) forms a non-Watson–Crick base pair with G1617 (equivalent to A1408), while A1709 is flipped out of the helix. Full size image The distortion of helix 44 by streptomycin also affects the orientation of A1408, which in the apo 30S structure is within hydrogen bonding distance of the tucked-in A1493 (ref. 12 ). An A1408G mutation confers streptomycin resistance to T. thermophilus [30] , and studies of an oligonucleotide analogue of the decoding site showed that this mutation slightly increases the thermal stability of the tucked-in conformation [31] , [32] . During decoding, C1407, A1408 and C1409 move laterally to accommodate the flipping out of A1492 and A1493. Streptomycin causes these bases to be displaced even further both in the absence and presence of ASL and mRNA, probably by restructuring bases C1490 to G1494 ( Fig. 4c ). Eukaryotic ribosomes contain a guanosine at the position equivalent to the bacterial A1408. In the recent crystal structure of the apo Tetrahymena thermophila 40S subunit (PDB entry 2XZM [33] , G1408 base-pairs with A1492 while A1493 adopts a flipped-out orientation ( Fig. 4d ). Both of these observations suggest that the A1408G mutation could confer resistance by stabilizing the tucked-in conformation of A1492, thereby counteracting the streptomycin-induced restructuring seen in Fig. 4c . Our observation that streptomycin stabilizes a bona fide decoding interaction of the near-cognate ASL Leu2 GAG is in excellent agreement with kinetic data of streptomycin-induced miscoding [6] . Streptomycin reduces the rate of GTP hydrolysis by EF-Tu for the cognate codon recognition and increases the rate for near-cognate recognition resulting in an almost complete loss of discrimination. Any distortion of the position of A1492 and A1493 is likely to reduce the efficiency of GTPase activation for cognate tRNAs. In contrast, the streptomycin-induced lateral displacement of A1492 and A1493 improves the accommodation of mismatched bases and consequently increases the rate of GTPase activation for near-cognate tRNAs. Crystal structures presented in this study reveal that the helix 45 tetraloop assumes two conformations. An engaged conformation in contact with helix 44 is seen with paromomycin, a disengaged conformation is seen with streptomycin and a disordered state with both conformations is seen in the apo 30S subunit. We recently reported a similar disengaged conformation in a crystal structure of the 30S subunit lacking post-transcriptional dimethylation of A1518 and A1519 in the helix 45 tetraloop [11] . Thus, disengagement of the helix 44–45 interaction is seen in two distinct conditions under which misreading occurs, in a methylation-deficient mutant and in the presence of streptomycin. A similar disengaged tetraloop conformation was modelled for PDB entry 1N34 (ref. 13 ) and entries 1I95, 1I96, and 1I97 (ref. 34 ). PDB entry 1N34 refers to the 30S structure in complex with near-cognate ASL Leu2 GAG (in the absence of paromomycin). In contrast, all 70S structures in the PDB were modelled with an engaged tetraloop conformation. This suggests that the formation of intersubunit bridge B2b between the 23S rRNA helix 69 and the 16S rRNA helices 24 and 45 stabilizes the helix 44–45 interaction. Together, these data indicate that the conformational dynamics of helix 45 would more likely contribute to the initiation phase of protein synthesis, before the formation of the 70S ribosome. In all structures with disengaged helix 45 presented here, we observed increased disorder in the conformation of helix 24a, which contacts helix 45 in its engaged conformation. Helix 24a contributes to tRNA coordination in the ribosomal P site and to positioning the mRNA E-site codon [35] . The two conformations of helix 45 could therefore indirectly affect the binding of tRNAs or modulate the interaction of IF3 with this region. Biochemical studies of ribosomes lacking helix 45 modifications (as a representative of a strongly disengaged conformation) indeed found reduced binding of fMet-tRNA fMet CAU and IF3 to 30S subunits [36] , defects in subunit association [37] and increased frameshifting [38] in support of a potential functional impact of the helix 45 dynamics on P site interactions during initiation. The increased dynamics of this interaction in the presence of streptomycin could explain its effects on the formation and stability of 70S initiation complexes [26] , [39] , [40] , [41] . In summary, the antibiotic streptomycin distorts the ribosomal decoding site in a previously unobserved manner. This reveals the high degree of conformational flexibility required for efficient tRNA decoding and also how streptomycin preferentially stabilizes near-cognate codon–anticodon interactions. These results provide a structural framework to understand streptomycin-induced ribosomal misreading of the genetic code. 30S subunit purification and crystallization 30S ribosomal subunits from T. thermophilus HB8 were purified and crystallized essentially as described [10] . ASL Phe GAA , ASL Leu2 GAG , ASL Ser GGA and the hexaU mRNA fragment were purchased from Dharmacon. Sequences for the ASLs (with anticodon sequences underlined) are GGGGAUU GAA AAUCCCC (ASL Phe GAA ), CUACCUU GAG GψGGUAG (ASL Leu2 GAG ) and CACGCCU GGA AAGψGUG (ASL Ser GGA ). 30S crystals were sequentially transferred to final buffer with 26% v/v 2-methyl-2,4-pentanediol for cryoprotection and soaks were performed in the final buffer supplemented with 200 μM of each ASL and mRNA and 800 μM paromomycin or 550 μM streptomycin for at least 1 week. Crystals were frozen in liquid nitrogen. Data collection and refinement Diffraction data were collected from a single crystal for all data sets. Data sets Apo, Strep, Par and MAP (mRNA, ASL Phe GAA , paromomycin) were collected with an ADSC 315 detector at beamline ID-24-C at the Advanced Photon Source in Argonne. Data sets Phe, Leu and Ser were collected with a Pilatus 6M detector at beamline X-25 at the National Synchrotron Light Source in Brookhaven. Diffraction data sets Apo, Strep, Par, and MAP were processed with the HKL2000 package [42] . All other data sets were processed with XDS [43] . Coordinates of the 30S subunit structure (PDB accession code 1J5E [12] ) with additional RNA and protein modifications were used for initial rigid body refinement with Phenix [14] for the Apo, Strep and Par data sets (PDB accession code 2VQE [44] ) was used for all other data sets). After simulated-annealing refinement, individual coordinates, three group B factors per residue and TLS parameters were refined. Potential positions of magnesium or potassium ions were compared with those in a high-resolution (2.5 Å) 30S subunit structure (PDB accession code 2VQE [44] ) in Coot [45] , and positions with strong difference density were retained. All magnesium atoms were replaced with magnesium hexahydrate. Water molecules located outside of significant electron density were manually removed. In both data sets with near-cognate ASLs, we modelled a second ASL molecule base paired to the extreme 3′-end of the 16S rRNA in a pseudo Shine-Dalgarno helix ( Supplementary Fig. S4 ). A similar refinement protocol was used for all data sets. Structure alignments were performed using the alignment algorithm of PyMol with the default 2σ rejection criterion and five iterative alignment cycles. All figures were produced with PyMOL [46] . Accession codes: Coordinates and structure factors have been deposited in the Protein Data Base under accession codes 4DR1 , 4DR2 , 4DR3 , 4DR4 , 4DR5 , 4DR6 , and 4DR7 for data sets Apo, Par, Strep, MAP, Sm-ASL Phe GAA -mRNA, Sm-ASL Leu2 GAG -mRNA, and Sm-ASL Ser GGA -mRNA, respectively. How to cite this article: Demirci, H. et al . A structural basis for streptomycin-induced misreading of the genetic code. Nat. Commun. 4:1355 doi: 10.1038/ncomms2346 (2013).